PKA regulatory subunits mediate synergy among conserved G-protein-coupled receptor cascades G-protein-coupled receptors sense extracellular chemical or physical stimuli and transmit these signals to distinct trimeric G-proteins. Activated Gα-proteins route signals to interconnected effector cascades, thus regulating thresholds, amplitudes and durations of signalling. Gαs- or Gαi-coupled receptor cascades are mechanistically conserved and mediate many sensory processes, including synaptic transmission, cell proliferation and chemotaxis. Here we show that a central, conserved component of Gαs-coupled receptor cascades, the regulatory subunit type-II (RII) of protein kinase A undergoes adenosine 3′-5′-cyclic monophosphate (cAMP)-dependent binding to Gαi. Stimulation of a mammalian Gαi-coupled receptor and concomitant cAMP-RII binding to Gαi, augments the sensitivity, amplitude and duration of Gαi:βγ activity and downstream mitogen-activated protein kinase signalling, independent of protein kinase A kinase activity. The mechanism is conserved in budding yeast, causing nutrient-dependent modulation of a pheromone response. These findings suggest a direct mechanism by which coincident activation of Gαs-coupled receptors controls the precision of adaptive responses of activated Gαi-coupled receptor cascades. Cells use versatile molecular signalling circuits to integrate and distinguish the quantity of extracellular signalling cues and to implement appropriate physiological responses. Cell surface plasma membrane receptors sense and the associated signal transducer guides the signal to adaptive intracellular effector circuits [1] , [2] . Adaptation is an essential feature of life, observed in a range of phenomena, including buffering of genetic variation in populations for the maintainance of homeostasis against perturbations in organisms and individual cells [3] , [4] . Signal transduction pathways often show adaptation to input signals, notably, allowing for sensing of chemical or light gradients over a wide range of concentrations or intensities as well as for polarization and direction sensing in chemotaxis [5] , [6] , [7] , [8] . Molecular mechanisms for adaptation are attributed to integral negative feedback circuits [8] that robustly convey the information sensed by cell surface receptors to accomplish the proper physiological response [2] , [9] , [10] . A key question about signalling is how sensitivities, amplitudes and durations of adaptive responses are controlled; particularly when coincident, potentially contradictory signals are received by a cell. An important class of signalling pathways in which to explore coincident signalling is among those coupled to the largest family of cell surface receptors, the G-protein-coupled receptor (GPCR) superfamily that are implicated in a large number of cellular processes, from light and hormone sensing to chemotaxis and memory consolidation [2] , [7] , [11] , [12] , [13] , [14] . Heterotrimeric G-proteins function as transducers of extracellular signals detected by GPCRs to intracellular effectors [2] . The adenosine 3′-5′-cyclic monophosphate (cAMP)-dependent protein kinase A (PKA) is the main and evolutionarily conserved cAMP effector of signal transduction in response to an assortment of hormones and physical stimuli [11] , [15] , [16] , [17] . In the canonical description of GPCR signalling, G-protein αs (Gαs)-coupled receptors activate adenylate cyclase (AC)-mediated synthesis of the second messenger cAMP, which in turn binds to PKA regulatory subunits (R), inducing dissociation of tetrameric R 2 :PKAc 2 (PKAc=PKA catalytic subunit) holoenzymes, resulting in active PKAc subunits ( Fig. 1a ) [15] , [17] , [18] . In contrast to the AC 'stimulatory' G-protein αs (Gαs)-coupled pathway, G-protein αi (Gαi)-coupled receptors 'inhibit' AC activities [19] . In addition various G-protein-dependent (for example, via Gαi:βγ) and G-protein-independent pathways link GPCRs to mitogen-activated protein kinase (MAPK) signalling cascades ( Fig. 1a ) [20] , [21] , [22] , [23] . The main cellular effectors of free diffusible cAMP are PKA R subunits. In addition to the function as cAMP sensors and inhibitor of PKAc activity, PKA R subunits bind to a variety of A kinase-anchoring proteins (AKAPs), thereby, facilitating spatial and temporal compartmentalization of PKA signalling [15] , [24] , [25] , [26] . 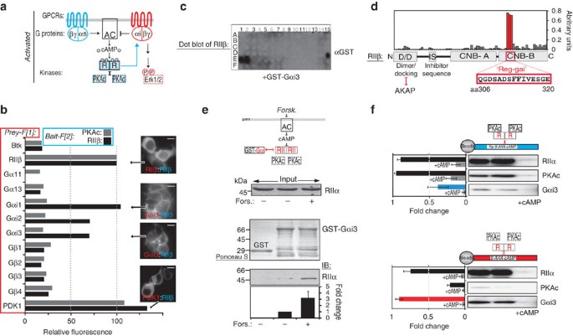Figure 1: PKA regulatory subunits form cAMP-dependent complexes with Gαi isoforms. (a) Schematic representation of GPCR cascades linked to cAMP turnover and MAPK activation. Gα-proteins modulate AC activities. Activation is shown by the arrows and inhibition is shown by T-bars. Blue arrow indicates novel connection of R subunits to G-protein-αi. Dotted lines indicate activated kinases (PKA subunits: R, PKAc; P stands for phosphorylated MAP kinase Erk1/2). (b) Fluorometric analysis of transiently transfected COS7 cells co-expressing PKA subunits as bait tagged with Venus-YFP PCA fragment[2] (RIIβ-F[2], PKAc-F[2]) with indicated prey proteins fused to F[1]. Fluorescence images of HEK293 cells co-expressing indicated protein pairs. Scale bar, 10 μm. (c) Spotted peptides (25 mers, 20 aa overlap) of RIIβ (aa1-25 spotted on A1, aa6-30 on A2 and so on) were overlaid with recombinant GST-Gαi3 followed by immunoblotting (IB). (d) Bar graph illustrates the densitometric quantification of the average ofn=3 dot blot experiments as shown inc. Red bars point to the sequence of the only binding interface of Reg:Gαi (red box; referred as 'Reggai peptide') in the illustrated modular structure of RIIβ. (e) Under basal conditions and following forskolin treatment (15 min, 100 μM) of HEK293 cells, we precipitated endogenously expressed RIIα with GST-Gαi3. Total RIIα and GST-Gαi3 are constant, but the quantity of co-precipitated GST-Gαi3:RIIα complexes increases following forskolin treatment. Fold enrichment of RIIα upon forskolin-mediated cAMP elevation is shown (normalized to levels of GST fusion proteins, ±s.e.m. ofn=3; pm, plasma membrane). (f) cAMP precipitation of endogenously expressed PKA complexes using 8-AHA-cAMP or Rp-8-AHA-cAMP immobilized to agarose resin from total brain lysates of mice. In the negative control experiment we added excess of cAMP (5 mM) to the brain lysates to mask the cAMP-binding sites in the R subunits for precipitation. We have performed densitometric quantification of RIIβ, PKAc and Gαi3 (normalized in each case to the most abundant protein) from the same immunoblot to compare complex formation and fold enrichment between holoenzyme (Rp-8-AHA-cAMP) and activated R complexes (8-AHA-cAMP). Results are presented as means ±s.e.m. from three independent experiments for each two independent precipitation. Treatments (italic) and readouts (red) are indicated. Figure 1: PKA regulatory subunits form cAMP-dependent complexes with Gαi isoforms. ( a ) Schematic representation of GPCR cascades linked to cAMP turnover and MAPK activation. Gα-proteins modulate AC activities. Activation is shown by the arrows and inhibition is shown by T-bars. Blue arrow indicates novel connection of R subunits to G-protein-αi. Dotted lines indicate activated kinases (PKA subunits: R, PKAc; P stands for phosphorylated MAP kinase Erk1/2). ( b ) Fluorometric analysis of transiently transfected COS7 cells co-expressing PKA subunits as bait tagged with Venus-YFP PCA fragment[2] (RIIβ-F[2], PKAc-F[2]) with indicated prey proteins fused to F[1]. Fluorescence images of HEK293 cells co-expressing indicated protein pairs. Scale bar, 10 μm. ( c ) Spotted peptides (25 mers, 20 aa overlap) of RIIβ (aa1-25 spotted on A1, aa6-30 on A2 and so on) were overlaid with recombinant GST-Gαi3 followed by immunoblotting (IB). ( d ) Bar graph illustrates the densitometric quantification of the average of n =3 dot blot experiments as shown in c . Red bars point to the sequence of the only binding interface of Reg:Gαi (red box; referred as 'Reggai peptide') in the illustrated modular structure of RIIβ. ( e ) Under basal conditions and following forskolin treatment (15 min, 100 μM) of HEK293 cells, we precipitated endogenously expressed RIIα with GST-Gαi3. Total RIIα and GST-Gαi3 are constant, but the quantity of co-precipitated GST-Gαi3:RIIα complexes increases following forskolin treatment. Fold enrichment of RIIα upon forskolin-mediated cAMP elevation is shown (normalized to levels of GST fusion proteins, ±s.e.m. of n =3; pm, plasma membrane). ( f ) cAMP precipitation of endogenously expressed PKA complexes using 8-AHA-cAMP or Rp-8-AHA-cAMP immobilized to agarose resin from total brain lysates of mice. In the negative control experiment we added excess of cAMP (5 mM) to the brain lysates to mask the cAMP-binding sites in the R subunits for precipitation. We have performed densitometric quantification of RIIβ, PKAc and Gαi3 (normalized in each case to the most abundant protein) from the same immunoblot to compare complex formation and fold enrichment between holoenzyme (Rp-8-AHA-cAMP) and activated R complexes (8-AHA-cAMP). Results are presented as means ±s.e.m. from three independent experiments for each two independent precipitation. Treatments (italic) and readouts (red) are indicated. Full size image Here we report that PKA regulatory subunits actively participate in Gαi signalling. We describe a novel and conserved mechanism through which cAMP-bound R subunits associate specifically with Gαi causing sensitization and increased amplitude and duration in response to Gαi-receptor activation. RII subunits form cAMP-dependent complexes with Gαi In a systematic screen for protein:protein interactions in mammalian COS7 cells, we identified novel interactions of PKA regulatory subunits type IIβ (RIIβ), but not PKAc subunits, with all the three isoforms of Gαi (Gαi 1,2,3 ) using a 'Venus' yellow fluorescent protein (YFP) protein-fragment complementation assay (PCA; Fig. 1b ; Supplementary Fig. S1a ) [27] , [28] , [29] . In addition, the phosphoinositide-dependent kinase 1 (PDK1) interacted with both RIIβ and PKAc, suggesting different modes of binding to PKA for this protein. Further, RIIβ:RIIβ and PDK1:RIIβ complexes were restricted to the cytosol, but Gαi:RIIβ complexes were localized at the plasma membrane, consistent with known localization of Gαi proteins ( Fig. 1b ). We confirmed the RIIβ:Gαi3 interaction in glutathione S -transferase (GST) pulldown assays. GST-RIIβ binds to endogenously expressed Gαi3 and GST-Gαi3 binds to purified RIIβ, suggesting that this interaction is direct ( Supplementary Fig. S1b,c ). In a dot blot screen of overlapping peptides derived from RIIβ (protein accession number: EAL24395 ), we identified a unique binding motif for Gαi3 within the evolutionarily conserved cyclic nucleotide binding domain B (CNB-B) and identified four amino acid (aa) positions required for binding to Gαi3: Asp 308, Phe 313, Phe 314 and Glu 317 ( Fig. 1c and d ; Supplementary Fig. S1d ). We next asked whether the binding of R subunits to Gαi could be cAMP-dependent and therefore actively mediated by GPCR signalling. First, in a GST pulldown assay from HEK293 cell lysates we confirmed the interaction of GST-Gαi3 and RIIα under basal conditions. However, pretreatment of cells with forskolin, a general activator of AC activity augments binding of endogenous cAMP-bound RIIα to GST-Gαi3 ( Fig. 1e ). Second, we applied total brain lysates of mice to 8-AHA-cAMP-coupled (precipitates 'active' R subunits) and Rp-8-AHA-cAMP-coupled (precipitates R:PKAc holoenzymes) agarose beads. Endogenous R subunits, bound to both types of agarose beads, co-precipitated endogenous Gαi3. In line with the observation from Figure 1e , we verified preferential binding of Gαi3 to endogenous and 'activated' R subunit complexes in vivo ( Fig. 1f ). These results were surprising, suggesting that in addition to cAMP binding to R subunits and mediating the dissociation of the R 2 :PKAc 2 holoenzyme, cAMP may mediate the active association of R subunit complexes to Gαi proteins. cAMP-bound R subunits modulate δOR-triggered Gαi activities To examine the potential role of R:Gαi complexes in GPCR signalling, we used a well-defined model cell, HEK293 cells stably expressing the exclusively Gαi-coupled δ-opioid receptor (δOR) [30] . First, we confirmed complex formation of R:Gαi3 in two independent cell lines under basal conditions, in HEK293 cells and in the osteosarcoma cell line U2OS, respectively ( Fig. 2a ; Supplementary Fig. S2a ). Next we determined how formation of cAMP-triggered R:Gαi complexes could effect δOR coupling to and activation of Gαi. For this purpose, we utilized bioluminescence resonance energy transfer (BRET)-based assays. The advantage of the first assay is that it directly reports on a known conformational rearrangement of the trimeric Gαi:βγ complex driven by ligand binding to a GPCR, coupled to the Gαi-protein complex ( Fig. 2b ) [31] . As expected, we observed that the δOR agonist SNC80 induced a decrease in BRET between Gαi1 and Gγ2, reflecting activation of the G-protein. However, and interestingly, direct activation of cAMP production by forskolin potentiated the Gαi1:Gγ2 conformational rearrangement resulting from receptor activation, suggesting that cAMP-mediated activation of PKA enhanced activation of Gαi, possibly via the formation of the R:Gαi1 complex. Forskolin treatment alone had no effect on the conformation of the trimeric G-protein complex ( Supplementary Fig. S2b ). Further, overexpression of RIIβ and the BRET sensor, but not of catalytically active PKAc, enhanced both SNC80 and SNC80+forskolin effects on the Gαi activation monitored by BRET ( Fig. 2b ). 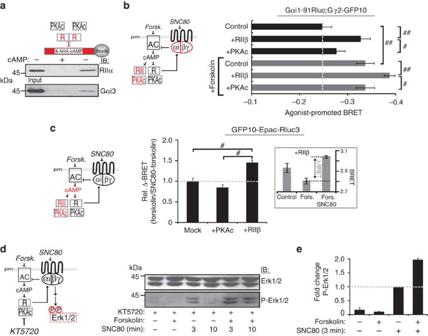Figure 2: cAMP-bound R subunit enhances ligand triggered Gαi activation and MAP kinase phosphorylation. (a) Endogenous R:Gαi3 complexes precipitated from HEK293 cells using 8-AHA-cAMP agarose (representative experiment ofn=3). (b) Conformational changes of trimeric G-proteins measured in δOR-HEK293 cells co-expressing the indicated BRET protein reporter pair and PKA subunits following stimulation with forskolin (100 μM, 15 min) and then by SNC80 (1 μM, 3 min; ±s.e.m.,n=3 independent experiments). (c) cAMP levels measured in δOR-HEK293 cells co-expressing the cAMP sensing EPAC BRET reporter and PKA subunits following stimulation with forskolin (50 μM, 12 min) and then SNC80 (1 μM, 6 min; ±s.e.m., representative experiment,n=3). Decrease in BRET ratio (Δ-BRET) indicates an increase in cAMP concentrationin vivo. Inset shows forskolin (±SNC80)-induced cAMP changes measured with EPAC-BRET in cells overexpressing RIIβ (±s.e.m.). (d) Effects of combinations of forskolin (100 μM, 15 min) and SNC80 (1 μM, minutes) on Erk1/2 phosphorylation in δOR-HEK293 cells; 60 min pretreatment with KT5720 (2 μM), representative experiment ofn=3. (e) Densitometric quantification of Erk1/2 phosphorylation upon SNC80/forskolin treatment, ±s.e.m. fromn=3. Statistical significance was assessed using a paired Student'st-test. Significance of individual results were determined at different levels as indicated with#and##(#P-values <0.05; ##P-values <0.01). Treatments (italic) and readouts (red) are indicated. Figure 2: cAMP-bound R subunit enhances ligand triggered Gαi activation and MAP kinase phosphorylation. ( a ) Endogenous R:Gαi3 complexes precipitated from HEK293 cells using 8-AHA-cAMP agarose (representative experiment of n =3). ( b ) Conformational changes of trimeric G-proteins measured in δOR-HEK293 cells co-expressing the indicated BRET protein reporter pair and PKA subunits following stimulation with forskolin (100 μM, 15 min) and then by SNC80 (1 μM, 3 min; ±s.e.m., n =3 independent experiments). ( c ) cAMP levels measured in δOR-HEK293 cells co-expressing the cAMP sensing EPAC BRET reporter and PKA subunits following stimulation with forskolin (50 μM, 12 min) and then SNC80 (1 μM, 6 min; ±s.e.m., representative experiment, n =3). Decrease in BRET ratio (Δ-BRET) indicates an increase in cAMP concentration in vivo . Inset shows forskolin (±SNC80)-induced cAMP changes measured with EPAC-BRET in cells overexpressing RIIβ (±s.e.m.). ( d ) Effects of combinations of forskolin (100 μM, 15 min) and SNC80 (1 μM, minutes) on Erk1/2 phosphorylation in δOR-HEK293 cells; 60 min pretreatment with KT5720 (2 μM), representative experiment of n =3. ( e ) Densitometric quantification of Erk1/2 phosphorylation upon SNC80/forskolin treatment, ±s.e.m. from n =3. Statistical significance was assessed using a paired Student's t -test. Significance of individual results were determined at different levels as indicated with # and ## ( # P -values <0.05; ## P -values <0.01). Treatments (italic) and readouts (red) are indicated. Full size image As activated Gαi is known to inhibit AC, we predicted that cAMP and R-mediated augmentation of Gαi activity should potentiate the δOR-mediated inhibition of AC and consequently decrease cAMP production. We tested this hypothesis using a BRET cAMP reporter based on the structure of the cAMP-regulated guanine nucleotide exchange factor (Epac) that undergoes conformational changes upon binding to cAMP. This assay enables accurate detection of in vivo cAMP levels indicated through a decrease of BRET [32] . We observed that overexpression of RIIβ, but not of PKAc, caused a further decrease in cAMP production when cells were treated with SNC80+forskolin compared with cells treated with forskolin alone ( Fig. 2c ). We next examined the potential function of R:Gαi complexformation on receptor-mediated activation of MAPK in mammalian cells [20] ( Figs 2 , 3 , 4 ) and budding yeast [33] ( Figs 5 and 6 ). We used the human δOR-HEK293 model for these experiments because they have the advantage that under basal condition and upon only Forskolin or only cAMP analogue treatments, no collateral effects on MAP kinase Erk1/2 activation are observed. As already known, the δOR-selective agonist SNC80 induces a transient increase of the Erk1/2 phosphorylation in δOR-HEK293 cells. Pretreatment with forskolin potentiated SNC80-induced Erk1/2 phosphorylation ( Fig. 2d,e ). These data support the notion that the cAMP-dependent R:Gαi complexes increase the sensitivity of this Gαi signalling pathway to δOR activation. The increase in sensitivity is distinct from activation through cross-talk in which a MAPK is activated by a Gαs-coupled receptor and dependent on PKA catalytic activity [22] , [34] . To exclude the possibility that PKA kinase activity could account for this potentiation, we pretreated cells with the PKA inhibitor KT5720 (unless noted otherwise, all subsequent experiments were carried out in the presence of this kinase activity inhibitor). The inhibition of catalytic PKA phosphotransferase activity did not prevent the forskolin-mediated potentiation of the MAPK activation ( Fig. 2d ). 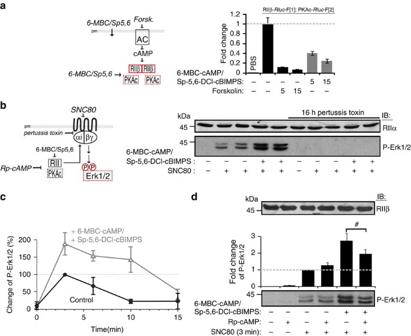Figure 3: cAMP-activated RII:Gαi enhances amplitude and duration of the MAP kinase pathway to δOR activation. (a–d) Effects of schematically indicated treatments (chemical modulators, overexpression) and combinations of 6-MBC-cAMP, Sp-5,6-DCl-cBIMPS (each 50 μM, 15 min) and the selective δOR agonist SNC80 (1 μM) on Erk1/2 phosphorylation (P-Erk1/2) in δOR-HEK293 cells. RII serves as loading control. (a) Time-dependent effects (in minutes) of combinations of Forskolin (50 μM) or 6-MBC-cAMP and Sp-5,6-DCl-cBIMPS (each 50 μM) on PKA type II holoenzyme dissociation measured from intact HEK293 cells stably expressing the indicatedRluc-PCA-based PKA reporter. (b) Effect of combinations of SNC80 (1 μM, 3 min) and 6-MBC-cAMP and Sp-5,6-DCl-cBIMPS on P-Erk1/2. Uncoupling of Gαi from the receptor through pretreatment with pertussis toxin (16 h, 100 ng ml−1; representative experiment). (c) Time-dependent effects of combinations of SNC80 and 6-MBC-cAMP, Sp-5,6-DCl-cBIMPS on P-Erk1/2; ±s.e.m. fromn=3. (d) Effect of pretreatment with Rp-cAMP (250 μM; 60 min) on P-Erk1/2. Densitometric quantification of Erk1/2 phosphorylation, ±s.e.m. fromn=3. Statistical significance was assessed using a paired Student'st-test. Significance of individual results were determined at different levels as indicated with#(#P-values <0.05). We confirmed that KT5720 inhibits PKA kinase activity under the conditions used in Figure 3 by monitoring the cAMP response element-binding protein (CREB) phosphorylation (activated independently of Gαi signalling; Supplementary Fig. S2c,d ). Figure 3: cAMP-activated RII:Gαi enhances amplitude and duration of the MAP kinase pathway to δOR activation. ( a–d ) Effects of schematically indicated treatments (chemical modulators, overexpression) and combinations of 6-MBC-cAMP, Sp-5,6-DCl-cBIMPS (each 50 μM, 15 min) and the selective δOR agonist SNC80 (1 μM) on Erk1/2 phosphorylation (P-Erk1/2) in δOR-HEK293 cells. RII serves as loading control. ( a ) Time-dependent effects (in minutes) of combinations of Forskolin (50 μM) or 6-MBC-cAMP and Sp-5,6-DCl-cBIMPS (each 50 μM) on PKA type II holoenzyme dissociation measured from intact HEK293 cells stably expressing the indicated R luc-PCA-based PKA reporter. ( b ) Effect of combinations of SNC80 (1 μM, 3 min) and 6-MBC-cAMP and Sp-5,6-DCl-cBIMPS on P-Erk1/2. Uncoupling of Gαi from the receptor through pretreatment with pertussis toxin (16 h, 100 ng ml −1 ; representative experiment). ( c ) Time-dependent effects of combinations of SNC80 and 6-MBC-cAMP, Sp-5,6-DCl-cBIMPS on P-Erk1/2; ±s.e.m. from n =3. ( d ) Effect of pretreatment with Rp-cAMP (250 μM; 60 min) on P-Erk1/2. Densitometric quantification of Erk1/2 phosphorylation, ±s.e.m. from n =3. Statistical significance was assessed using a paired Student's t -test. Significance of individual results were determined at different levels as indicated with # ( # P -values <0.05). 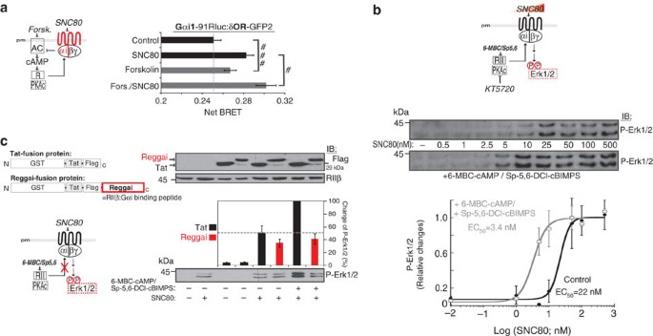Figure 4: cAMP-activated RII:Gαi enhances sensitivity of the MAP kinase pathway to δOR activation. Effects of schematically indicated treatments (chemical modulators, hybrid fusion proteins) and combinations of forskolin (100 μM, 15 min), 6-MBC-cAMP, Sp-5,6-DCl-cBIMPS (each 50 μM, 15 min) and varying concentrations of the selective δOR agonist SNC80 (3 min) on G-protein coupling and Erk1/2 phosphorylation (P-Erk1/2) in δOR-HEK293 cells. (a) Conformational changes of Gαi1-protein coupling to δOR measured in HEK293 cells co-expressing indicated BRET protein reporter pairs following stimulation with forskolin (100 μM, 15 min) and then by SNC80 (1 μM, 3 min; ±s.e.m.,n=3 independent experiments). Statistical significance was assessed using a paired Student'st-test. Significance of individual results were determined as indicated with#and###(#P-value <0.05;###P-value <0.001). (b) Dose-dependent effects of combinations of SNC80 (3 min) and 6-MBC-cAMP and Sp-5,6-DCl-cBIMPS on P-Erk1/2 following pretreatment with KT5720 (60 min, 2 μM), ±s.e.m. fromn=3. (c) Domain structure for the Reggai peptide fused to GST-TAT-Flag peptide. Treatments of δOR-HEK293 cells with either TAT control or the Reggai fusion peptides (each ~3 μM; 30 min) on P-Erk1/2 are shown; ±s.e.m. fromn=4. RIIβ serves as loading control. (b, c) Pretreatment with KT5720 (60 min, 2 μM). Treatments (italic) and readouts (red) are indicated. Full size image Figure 4: cAMP-activated RII:Gαi enhances sensitivity of the MAP kinase pathway to δOR activation. Effects of schematically indicated treatments (chemical modulators, hybrid fusion proteins) and combinations of forskolin (100 μM, 15 min), 6-MBC-cAMP, Sp-5,6-DCl-cBIMPS (each 50 μM, 15 min) and varying concentrations of the selective δOR agonist SNC80 (3 min) on G-protein coupling and Erk1/2 phosphorylation (P-Erk1/2) in δOR-HEK293 cells. ( a ) Conformational changes of Gαi1-protein coupling to δOR measured in HEK293 cells co-expressing indicated BRET protein reporter pairs following stimulation with forskolin (100 μM, 15 min) and then by SNC80 (1 μM, 3 min; ±s.e.m., n =3 independent experiments). Statistical significance was assessed using a paired Student's t -test. Significance of individual results were determined as indicated with # and ### ( # P -value <0.05; ### P -value <0.001). ( b ) Dose-dependent effects of combinations of SNC80 (3 min) and 6-MBC-cAMP and Sp-5,6-DCl-cBIMPS on P-Erk1/2 following pretreatment with KT5720 (60 min, 2 μM), ±s.e.m. from n =3. ( c ) Domain structure for the Reggai peptide fused to GST-TAT-Flag peptide. Treatments of δOR-HEK293 cells with either TAT control or the Reggai fusion peptides (each ~3 μM; 30 min) on P-Erk1/2 are shown; ±s.e.m. from n =4. RIIβ serves as loading control. ( b, c ) Pretreatment with KT5720 (60 min, 2 μM). Treatments (italic) and readouts (red) are indicated. 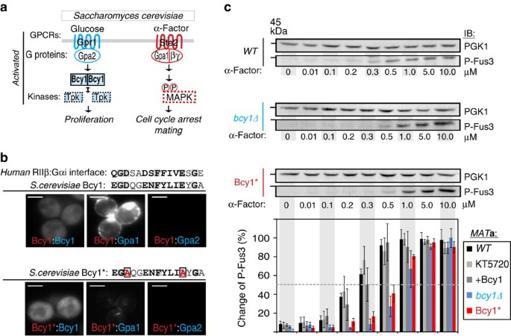Figure 5: Conservation of cAMP-dependent modulation of MAP kinase signallingviaR:Gαi (Bcy1:Gpa1) in yeast. (a) Schematic illustration of the conserved components of glucose and α-factor triggered signalling pathways inS. cerevisiaeand their functional/morphological effects. (b) Fluorescence images of yeast cells expressing the indicated protein pairs fused to Venus YFP PCA F[1] and F[2] reporter protein fragments. Alignment of the human RIIβ:Gαi interface ('Reggai peptide') to yeast homologue Bcy1 (grey box=conservation, bold=conserved substitutions, grey=semi-conserved substitution). Indication of double mutations (in red) in the conserved sequence regions ofBcy1. Scale bar, 5 μm. (c) Dose-dependent effects of α-factor exposure (15 min) on phosphorylation of MAP kinase Fus3 in followingMATastrains:WT,WT+KT5720,WT+Bcy1,bcy1Δandbcy1Δ+Bcy1* (in the presence of glucose detected by IB using an anti-phospho MAPK antibody). Densitometric quantification of the Fus3 phosphorylation upon dose-dependent α-factor treatment normalized on the loading control PGK1, ±s.d. fromn=3. Full size image Figure 5: Conservation of cAMP-dependent modulation of MAP kinase signalling via R:Gαi (Bcy1:Gpa1) in yeast. ( a ) Schematic illustration of the conserved components of glucose and α-factor triggered signalling pathways in S. cerevisiae and their functional/morphological effects. ( b ) Fluorescence images of yeast cells expressing the indicated protein pairs fused to Venus YFP PCA F[1] and F[2] reporter protein fragments. Alignment of the human RIIβ:Gαi interface ('Reggai peptide') to yeast homologue Bcy1 (grey box=conservation, bold=conserved substitutions, grey=semi-conserved substitution). Indication of double mutations (in red) in the conserved sequence regions of Bcy1 . Scale bar, 5 μm. ( c ) Dose-dependent effects of α-factor exposure (15 min) on phosphorylation of MAP kinase Fus3 in following MAT a strains: WT , WT +KT5720, WT +Bcy1, bcy1Δ and bcy1Δ +Bcy1* (in the presence of glucose detected by IB using an anti-phospho MAPK antibody). Densitometric quantification of the Fus3 phosphorylation upon dose-dependent α-factor treatment normalized on the loading control PGK1, ±s.d. from n =3. 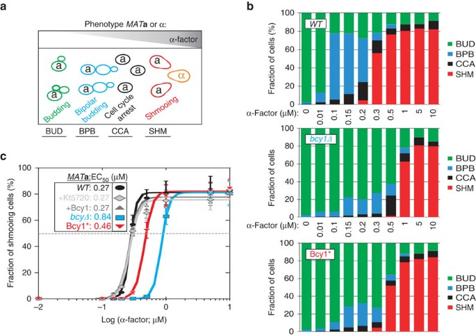Figure 6: Impact of cAMP-dependent modulation of MAP kinase signalling on morphological changes in yeast. (a) Schematic illustration of morphological changes upon activation of the α-factor pheromone pathway inS. cerevisiae. (b) Quantification of the phenotypic (morphological) consequences of dose-dependent α-factor exposure (3–4 h) inwildtype(WT),bcy1Δstrains and in thebcy1Δstrain expressing Bcy1* in the presence of glucose (BUD, budding; BPB, bipolar budding; CCA, cell cycle arrest; SHM, Shmooing). (c) Dose–response curves with indicated α-factor EC50concentrations for shmooing under the indicated conditions in the yeastMatastrainsWT,WT+KT5720,WT+Bcy1,bcy1Δandbcy1Δ+Bcy1*; ±s.d. from three independent experiments. Full size image Figure 6: Impact of cAMP-dependent modulation of MAP kinase signalling on morphological changes in yeast. ( a ) Schematic illustration of morphological changes upon activation of the α-factor pheromone pathway in S. cerevisiae . ( b ) Quantification of the phenotypic (morphological) consequences of dose-dependent α-factor exposure (3–4 h) in wildtype ( WT ), bcy1Δ strains and in the bcy1Δ strain expressing Bcy1* in the presence of glucose (BUD, budding; BPB, bipolar budding; CCA, cell cycle arrest; SHM, Shmooing). ( c ) Dose–response curves with indicated α-factor EC 50 concentrations for shmooing under the indicated conditions in the yeast Mat a strains WT , WT +KT5720, WT +Bcy1, bcy1Δ and bcy1Δ +Bcy1*; ±s.d. from three independent experiments. Full size image cAMP-RII subunits modulate δOR-triggered Gαi activities We next asked whether cAMP-bound forms of distinct PKA regulatory subunits type I (RI) or R type II (RII) increase the sensitivity of Gαi-mediated δOR signalling [15] . We thus directly activated endogenous PKA with combinations of membrane permeable cAMP analogues that bind selectively to the CNB-A or CNB-B of RI or RII [35] , [36] . We first determined the concentration- and time-dependent effects of each cAMP analogue on RII:PKAc dissociation in intact cells (using a Renilla luciferase ( R luc)-based PKA reporter assay [29] ; Fig. 3a ; Supplementary Fig. S3 ). Maximally active RI subunit cAMP analogues (8-PIP-cAMP, 2-Cl-8-MA-cAMP) had no effect, but the RII subunit-binding analogues (6-MBC-cAMP, Sp-5,6-DCl-cBIMPS [35] , [36] ) potentiated the amplitude and duration of SNC80-induced Erk1/2 phosphorylation ( Fig. 3b,c ; Supplementary Figs S3c,4a ). These observed effects occurred through Gαi signalling as pretreatment of cells with pertussis toxin, which uncouples Gαi from the receptor, prevented both receptor and cAMP analogue-potentiated Erk1/2 phosphorylation ( Fig. 3b ). We next asked whether RII binding to Gαi may enhance sensitivity of Gαi-coupled receptor signalling by somehow shifting Gαi to its active, GTP-bound state. We used an antibody to selectively precipitate GTP-loaded Gαi in untreated, SNC80 or SNC80 plus RII-specific cAMP-analogue-treated δOR-HEK293 cells. By immunoblotting (IB) with the isoform selective Gαi3 antibody we observed elevated levels of immunoprecipitated GTP-Gαi3, following both RII and δOR activation ( Supplementary Fig. S4b ). Exclusive treatment with RII-specific cAMP-analogues shows no activation of Erk1/2 in HEK293 cells (see below, Fig. 4b ). These results, together with our observation of enhanced conformation change of Gαi:βγ complex under the same conditions ( Fig. 2b ), suggest that the active GTP–Gαi complex is favoured when bound to cAMP-RII:Gαi following Gαi-coupled receptor activation. Our results suggest that preventing cAMP-triggered PKA dissociation and hence formation of RII:Gαi complexes would prevent Gαi-coupled receptor signal augmentation by cAMP. To test this prediction, we used the cAMP analogue Rp-cAMP, an inhibitor of PKA holoenzyme dissociation. Pretreatment with Rp-cAMP decreased SNC80+RII subunit activator (6-MBC-cAMP, Sp-5,6-DCl-cBIMPS) and SNC80+forskolin-mediated Erk1/2 phosphorylation ( Fig. 3d ) to a similar extent as it prevented PKA holoenzyme dissociation ( Supplementary Fig. S4c,d ). cAMP-RII:Gαi complexes modulate ligand sensitivity We next tested whether the induction of cAMP-'activated' RII:Gαi complexes affect receptor:G protein coupling. First, we performed a BRET assay that reports directly on Gαi1 coupling to δOR in response to agonist binding to the GPCR [30] , [31] . We observed that forskolin potentiated the SNC80-induced increase in BRET between δOR and Gαi1 ( Fig. 4a ), which is consistent with the idea that the formation of the RII:Gαi complex potentiates the receptor-mediated activation of Gαi1. Moreover, a dose–response of the δOR agonist SNC80-mediated ERK1/2 phosphorylation following pretreatment with the selective PKA phosphotransferase inhibitor KT5720 performed in the presence and absence of RII subunit-specific cAMP analogues showed a significant, sevenfold increase in sensitivity of the MAPK pathway to stimulation ( Fig. 4b ). To test whether direct disruption of the RII:Gαi complex would prevent cAMP-dependent sensitization of Gαi to receptor activation, we created a membrane-permeable peptide competitive antagonist of RII:Gαi binding based on the Gαi3 binding motif that we identified in RII ( Fig. 1c,d ). Coding sequence for this peptide was fused to that of the membrane-permeant HIV TAT peptide and expressed in and purified from Escherichia coli [37] . Treatment of cells with this peptide (we call Reggai) prevented the potentiation of SNC80-mediated Erk1/2 phosphorylation by RII subunit-specific cAMP analogues ( Fig. 4c ). A TAT control peptide had no effect. These data highlight that formation of cAMP-dependent RII:Gαi complexes are required for the transmission of signal from Gαs- to activated Gαi-cascades. cAMP-RII modulation of Gαi is conserved in budding yeast The evolutionary conservation of PKA R subunits and notably of two critical aa's for interaction in the Reggai sequence, Asp 308 and Glu 317 ( Fig. 5b ; Supplementary Fig. S1d ), prompted us to evaluate whether the cAMP-bound R subunit-mediated modulation of Gαi signalling is also conserved in yeast. The budding yeast Saccharomyces cerevisiae (S. cerevisiae) has homologues of the mammalian signalling components for both PKA and MAPK pathways downstream of GPCRs. Yeast express the glucose-sensing Gαs-coupled receptor Gpr1 and in the MAT a haploid strain, the Ste2 pheromone receptor, which is Gαi-coupled ( Fig. 5a ) [17] , [38] . The signalling counterpart to the Gαi:βγ-MAPK cascade in S. cerevisiae is activated by the mating pheromone α-factor (in MAT a haploid cells), resulting in a distinct morphogenic 'shmoo' response ( Figs 5a and 6a,b ) [33] . We first tested for interactions of the single Gαi and Gαs homologues (Gpa1 and Gpa2) with the single yeast PKA R subunit Bcy1, using the Venus YFP PCA and observed that Gpa1, but not Gpa2, interacts with Bcy1 in a complex at the plasma membrane ( Fig. 5b ; Supplementary Fig. S5 ). These results are consistent with our observations in mammalian cells ( Fig. 1b ). Furthermore, point mutations of homologous Asp 308 and Glu 317 residues in the Reggai binding motif of Bcy1 decreased the interaction of Bcy1 with Gpa1, but did not affect the Bcy1:Bcy1 or Bcy1:Tpk2 (Tpk=PKAc) complexes ( Fig. 5b ; Supplementary Fig. S5 ). Finally, we observed that mammalian RIIβ and Gαi3 interacted with the yeast R subunit Bcy1 ( Supplementary Fig. S6 ). These results suggest that the specific R:Gαi interaction has been conserved for at least 1.5 billion years since Metazoa and Fungi lineages separated [39] . We next examined the role of Bcy1 on downstream pheromone signalling, including activation of the yeast MAPK homologue Fus3 phosphorylation and the 'shmoo' response [33] in the presence of the trigger for cAMP-production, glucose. We observed an approximately threefold decrease in sensitivity to α-factor-induced Fus3 phosphorylation and 'shmoo' response (EC 50 right shift) in an isogenic knockout of the bcy1 gene ( bcy1Δ ) ( Fig. 5c lower panel, Fig. 6c ). These data correlate with the observation that in mammalian cells activation of PKA RII shifts the EC 50 curve of Gαi-coupled receptor activation to the left ( Fig. 4b ). Expression of a Reggai-binding motif mutant of Bcy1 (=Bcy1*) expressed in the bcy1Δ strain produced an intermediate decrease in both Fus3 phosphorylation (twofold) and also the 'shmoo' response (1.6-fold). Overall, the reduced MAP kinase activation and 'shmoo' response in yeast resulting in a EC 50 shift of α-factor to higher concentration indicates that, as in mammalian cells, the yeast R subunit Bcy1 potentiated the Gαi:βγ-mediated MAPK pathway ( Figs 5c and 6 ). However, we observed no impact of Bcy1 overexpression on MAPK activation and on the shmooing response, suggesting that Bcy1 is already highly expressed in yeast and that the pathway is less sensitive to overexpression. Further, consistent with our model, the PKA inhibitor KT5720 had no effect on MAPK phosphorylation or the shmoo response ( Fig. 5c lower panel, Fig. 6c ). In summary, data presented in Figures 4 , 5 , 6 support our argument for an evolutionarily conserved function of R subunits in regulating the sensitivity of Gαi-coupled signalling responses (shift of EC 50 curves). Application of the Reggai peptide in mammalian cells ( Fig. 4c ) and mutational modification of the same motif in budding yeast R subunits (Bcy1; Figs 5c and 6b,c ) suggests a conserved mechanism for cAMP-bound R subunits to modulate Gαi signalling. Over the past 40 years, the canonical view of GPCR cascades regulating cAMP synthesis has placed the PKA R subunit in the role of inhibiting PKAc subunit activity [15] , [16] , and more recently, localizing specific signalling complexes to subcellular locations through AKAP scaffolding proteins [24] , [26] . We now report the discovery that cAMP-activated R subunits (functioning as pivotal component of Gαs-coupled receptor cascades) directly bind to and modulate Gαi-coupled receptor signalling ( Fig. 7 ). In contrast to AKAP binding via the N-terminal docking domain of R subunits, the cAMP-dependent interaction between RII:Gαi is mediated by the flexible, cAMP-binding CNB domain, which is conserved in all organisms, except in plants [40] . We describe how this dynamic binary interaction provides a simple means to control sensitivity, amplitude and duration of adaptive signalling responses. 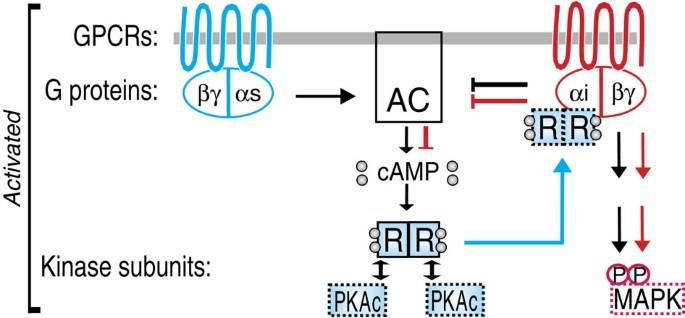Figure 7: Schematic representation of the role of R subunits in Gαi signalling. Activation is shown by arrows and inhibition is shown by T-bars. The blue arrow indicates the novel binary protein:protein interaction between the PKA regulatory subunit (R) and the Gαi; PKAc stands for PKA catalytic subunit. Dotted lines indicate activated kinases or kinase subunits. The red arrows indicate the cAMP-bound R-subunit-mediated augmentation of receptor triggered Gαi activities: cAMP elevation promotes dissociation of the PKA heterotetramer (R2:PKAc2) and recruitment of R subunits to Gαi, which amplifies the duration and amplitude of Gαi-coupled receptor triggered signalling responses along with sensitization of GPCR-mediated signal transmission. This mechanism elevates ligand triggered MAPK responses (phosphorylation [P] of Erk1/2 in mammalian cells and of Fus3 inS.cerevisiae) and inhibition of ACs. Figure 7: Schematic representation of the role of R subunits in Gαi signalling. Activation is shown by arrows and inhibition is shown by T-bars. The blue arrow indicates the novel binary protein:protein interaction between the PKA regulatory subunit (R) and the Gαi; PKAc stands for PKA catalytic subunit. Dotted lines indicate activated kinases or kinase subunits. The red arrows indicate the cAMP-bound R-subunit-mediated augmentation of receptor triggered Gαi activities: cAMP elevation promotes dissociation of the PKA heterotetramer (R 2 :PKAc 2 ) and recruitment of R subunits to Gαi, which amplifies the duration and amplitude of Gαi-coupled receptor triggered signalling responses along with sensitization of GPCR-mediated signal transmission. This mechanism elevates ligand triggered MAPK responses (phosphorylation [P] of Erk1/2 in mammalian cells and of Fus3 in S.cerevisiae ) and inhibition of ACs. Full size image We present a detailed molecular description of how activated R subunits in yeast and mammalian cells directly control Gαi-mediated activation of MAPK responses. In the yeast model, the function of the R:Gαi interaction is clear. Diploid yeast undergoes meiosis when starved and haploids mate when nutrients become available. Glucose, the preferred carbon source of yeast, activates a Gαs-coupled receptor and in turn cAMP synthesis and PKA activation. It, thus, follows that the modulation of pheromone sensitivity that we observe is mediated by R subunit binding to Gαi and serves to sensitize the pheromone response to the fact that the best carbon source is available [17] . In mammalian cells, the phosphotransferase-independent function of cAMP-bound R subunits reported here will need to be understood in the context of known GPCR signalling dynamics [11] , [12] , [41] , [42] , [43] . First, ACs and GPCRs are themselves targets of receptor-activated kinases that control ligand sensitivity and turnover and can lead to the activation of distinct G-protein pathways (switch from primary G-protein-coupling from Gαs to Gαi), as observed for human β 2 -adrenergic receptor activation [19] , [44] , [45] , [46] . This is distinct from the mechanism we describe here, in which a constituent of Gαs-coupled receptor signalling directly functions on Gαi-coupled receptor signalling. Second, the distinct sites of protein:protein interaction for AKAPs and Gαi ( Fig. 1d ) suggest that cAMP-activated RII subunits bring AKAPs into proximity of Gαi and its receptor/effectors (see also below, 'fifth'), further organizing compartmentalized signalling complexes [11] , [22] , [24] , [26] , [44] . Third, recently the mammalian E3 ubiquitin ligase praja2 has been shown to target R subunits for degradation in a cAMP-dependent manner and thus, could change the degree of sensitivity of Gαi-coupled receptor signalling to cAMP-RII modulation of Gαi [26] . Fourth, the mechanism we propose creates a negative feedback loop, resulting in downregulation of cAMP synthesis via Gαi activation and AC inhibition. This negative feedback could cause adaptation to Gαi-coupled signalling itself and also function in concert with other feedback circuits to generate cAMP oscillations that couple to other, for example, calcium and MAPK oscillators, and may control spatial and temporal signalling by PKA [25] , [47] . Fifth, beyond MAPK and AC modulation, Gαi signalling has a broad spectrum of protein effectors, linking Gαi to a variety of diverse cellular processes, for example, those involved in development and autophagy [46] . It will, thus, be interesting to explore how co-incident modulation of Gαi signalling by Gαs-generated cAMP-RII may function in these pathways. Gαs-mediated control of Gαi signalling via cAMP-RII could be a common mechanism of GPCR-mediated adaptive signalling in, as examples, chemotaxis or long-term potentiation in neuronal circuits [7] , [13] , [14] , [44] , [47] , [48] , [49] . Chemokine and most neurotransmitter receptors mediate adaptive responses and are coupled to Gαi, but Gαs-proteins upstream of its main effector PKA are mostly activated by metabolic hormones or autonomic neurotransmitters [50] . In this context, we confirmed complex formation of 'activated' PKA R subunit complexes and G-protein-αi3 in mammalian brains under physiological conditions ( Fig. 1f ). It will be interesting to explore how the mechanism we report contributes to controlling sensitivity to signals and chemotactic responses or neural information processing where a neuron responds to one synapse that releases a Gαi-coupled receptor activator, while another simultaneously releases a Gαs-coupled receptor binding hormone [14] , [49] . Finally, our results have at least four implications to understanding GPCR and PKA pharmacology. First, the fact that Gαi signalling sensitivity is increased by Gαs-coupled receptor signalling means that the sensitivity of Gαi-coupled receptor signalling processes could be increased by drugs that positively function on Gαs-coupled receptors ( Fig. 4a,b ) [51] . At the same time, the efficacy of Gαi-coupled receptor agonists/antagonists could be modified by treatment with Gαs-coupled receptor drugs. There are currently compounds in clinical trials for diseases of aberrant cell proliferation such as cancers (for example, compounds functioning on Gαi-coupled CXCR4 and Smoothened receptors), and it would be interesting to test whether Gαs-coupled GPCR agonists alter the efficacies of these compounds [52] , [53] , [54] . Moreover, distinct mechanisms have been proposed to explain how cAMP regulates cell-type-specific MAPK signalling, which modulates cell growth and proliferation, either positively or negatively [55] . For instance, human endocrine tumours have mitogenic MAPK activities caused by activating mutations of Gαi2 (refs 20 , 23 , 56 , 57 , 58 ). Finally, cAMP analogues are being used to treat memory deficiencies caused by neurodegenerative diseases [59] . The actions of these compounds will need to be considered in light of the mechanism that we have discovered. The Reggai peptide we report here may, itself prove a useful lead for development of drugs that modulate sensitivity of Gαi-coupled, for example, neurotransmitter receptors. Antibodies Antibodies used were anti-RIIβ (BD Bioscience, #610626, 1:2000), anti-RIIα (BD Bioscience, #612242, 1:2000), anti-PKAcα (BD Bioscience, #610981, 1:2000), anti-Gαi3 (Santa Cruz, #sc-262, 1:200), anti-active Gαi antibody (New East Biosciences, #26901, 1 microgram/precipitation), anti-Erk1/2 (Cell Signaling, #9102, 1:2000), anti-phospho-Erk1/2 (Cell Signaling, #9101, 1:2000), anti-CREB (Cell Signaling, #9104, 1:1000), anti-phospho-Serine133-CREB (Cell Signaling, #9198, 1:1000), anti-GFP (Roche, #11814460001, 1:2000, anti-Flag (Sigma, #F3165, 1:2000) and anti-GST (Sigma, #G1160, 1:1000). Construction of plasmids Venus YFP PCA expression vectors and fusion constructs The PKA regulatory subunit (rat, RII β) and the PKA catalytic subunit (mouse, PKAc α) were subcloned into the 5′-end to the Venus YFP PCA fragments, referred to here as N-terminal fragment (1–158 aa; F[1]) and the C-terminal fragment (159–239 aa; F[2]) as previously described [27] , [28] , [29] . To screen for interacting proteins, we generated plasmids designed to serve as expression and destination vectors for lambda recombinase subcloning of mouse cDNAs harboured in Gateway-ready entry vectors (unpublished results). Venus YFP PCA fragments were subcloned into a pcDNA 3.1 expression vector with the appropriate Gateway reading frame cassette to generate the C- and N-terminal destination vectors for each PCA fragment. cDNAs of interest were subcloned into these destination vectors with LR (lambda recombinase) clonase as recommended by the manufacturer (Invitrogen Corporation). GST fusion protein constructs. We constructed a fusion protein consisting of Gαi3 and GST to be used in GST pulldown experiments and dot blot analysis. The cDNA for G α i3 was amplified from rat heart Marathon-Ready cDNA (BD Biosciences) by PCR and cloned into the multiple cloning site of the GST expression vector pGEX-5X-1 via Eco RI/ Xho I. The GST–RIIβ construct was kindly provided by E. Klussmann (FMP-Berlin, Free University Berlin). Oligos coding for the 15 amino acids of the Reggai peptide were cloned into the multiple cloning site of pGEX-4T-2 ( via Eco RI/ Xho I) flanked upstream with the sequences for GST , Tat and Flag antigenic peptide tag [37] . All GST fusion proteins were expressed in E. coli (strain BL21). Induction, cell lysis and affinity purification of fusion proteins were performed as recommended by the supplier of the pGEX vectors (GE Healthcare). Fluorometric analysis of Venus-PCA-tagged proteins COS7 cells grown in 12-well plates were co-transfected with the Venus YFP PCA expression vectors (pcDNA3.1) coding for prey-F[1] and/or bait-F[2] using FuGENE6 reagent (Roche). Fluorometric analysis and imaging have been performed as previously described [27] , [28] , [29] . For localization of protein–protein interactions in S. cerevisiae , we utilized the same variants of Venus YFP PCA fragments as described above. We co-transformed MAT a (strain BY4741) strains of S.cerevisiae with plasmid p413 (for F[1]; ADH promotor) and plasmid p415 (for F[2]; ADH promotor) encoding the following Venus YFP PCA fusions (Bcy1-F[1], Bcy1-F[2], Bcy1*-F[1], Bcy1*-F[2], Tpk2-F[1], Gpa1-F[2] and Gpa2-F[2]). Positive clones were selected on the synthetic complete media lacking Histidine (His) and Leucine (Leu). Cells were grown in low-fluorescent media, and images were taken using a Nikon Eclipse TE2000U inverted microscope (Nikon) with ×60 objective and YFP filter cube (41028, Chroma Technologies). Images were captured with a CoolSnap CCD camera (Photometrics) using Metamorph software (Molecular Devices). We quantified the fluorescence intensities from individual cells using the ImageJ software. SPOT synthesis and overlay experiments Overlapping peptides, either of RIIβ or peptides-containing substitutions of conserved amino acids in the Reggai sequence, were SPOT synthesized on distinct coordinates of a cellulose membrane. Membranes were overlaid with recombinant GST-Gαi3 (10 μg ml −1 blocking buffer). Interactions were detected with anti-GST and secondary horseradish peroxidase antibodies by a procedure identical to IB. cAMP agarose protein precipitation assays HEK293, U2OS cells and total brains of mice were homogenized using a Potter S (B. Braun Biotech International) with 15 strokes. We clarified the lysate (13,000 r.p.m., 15 min) and precipitated the R-subunit-associated protein complexes with PKA-selective 8-AHA-cAMP agarose and Rp-8-AHA-cAMP agarose resin (Biolog, #D014, #M012) for 2 h at 4 °C. As negative control experiment we added excess of cAMP (5 mM) to lysates to mask the cAMP-binding sites in the R subunits for precipitation. Resin-associated proteins were washed four times with lysis buffer and eluted with Laemmli sample buffer. Equal amount of protein were subjected to polyacrylamide gel electrophoresis followed by IB. We performed densitometric quantification of RIIβ, PKAc and Gαi3 (in each case, normalized to the most abundant precipitated protein) from the same immunoblot ( n =3) to compare complex formation and fold enrichment between holoenzyme (precipitated with Rp-8-AHA-cAMP) and activated R complexes (precipitated with 8-AHA-cAMP). Bioluminescence resonance energy transfer measurements δOR-HEK293 cells were transiently transfected with Gαi1 with the R luc inserted at aa position 91 and the ultraviolet-shifted GFP variant GFP10 (substitutions: P64L, S147P and S202P) fused to the C-terminus of Gγ2 or the ultraviolet-shifted variant GFP2 (substitution: F64L) fused to the C-terminus of the δOR. In overexpression studies, we co-expressed RIIβ or PKAc. For cAMP measurements, we co-expressed the cAMP-sensing Epac in vivo cAMP reporter assay GFP10-Epac-Rluc3 ( R luc3= R luc variant with following substitutions: A55T, C124A and M185V) and either RIIβ or PKAc. Forty-eight hours after transfection, cells were treated with combinations of forskolin (100 μM) and SNC80 (1 μM), washed twice with PBS, detached with PBS plus 5 mM EDTA and resuspended in PBS plus 0.1% (w/v) glucose. Equal amount of cells (100,000 cells per well) were distributed in a 96-well microtitre plate (Optiplate, PerkinElmer, Life Science). Total fluorescence and bioluminescence were evaluated for each well using a FlexStation II (Molecular Devices) and Mithras LB 940 (Berthold Technologies), respectively. uvGFP fluorescence was excited at 400 nm and read at 515 nm. Fluorescence values were corrected by subtracting the autofluorescence of cells that do not expressed uvGFP. BRET between R luc and GFP2 or GFP10 was measured after the addition of 5 μM R luc substrate DeepBlueC (bisdeoxycoelenterazine, PerkinElmer, Life Science). BRET signals were derived from the emission detected with the energy-acceptor filter (515±15 nm; GFP2/10) divided by the emission detected with the energy-donor filter (410±40 nm; R luc/ R luc3). MAPK phosphorylation assay Mammalian cells δOR-HEK293 cells were grown in 12- or 24-well plate formats. Either 24 or 48 h after splitting or co-transfection in overexpression studies, confluent cells were treated with inhibitors (KT5720 for 60 min, pertussis toxin for 16 h), chemical modulators (forskolin, 6-MBC-cAMP, Sp-5,6-DCl-cBIMPS, Sp-8-PIP-cAMPs, 2-Cl-8-MA-cAMP (all for 15 min) or Rp-cAMP for 60 min) and/or the δOR ligand SNC80 (for 3, 6, 10 or 15 min). cAMP analogues were purchased from Biolog (6-MBC-cAMP, #M012; Sp-5,6-DCl-cBIMPS, #D014; Sp-8-PIP-cAMPs, #P005, 2-Cl-8-MA-cAMP, #C080; Rp-cAMP, # A002S) [35] , [36] . Following treatments at 37 °C, the reactions were stopped by direct addition of Laemmli sample buffer. Equal amount of protein were subjected to polyacrylamide gel electrophoresis followed by IB. Yeast cells S . cerevisiae MAT a cells (strain BY4741) were grown overnight to saturation in complete or appropriate selective medium (for example, synthetic complete medium lacking His and Leu). Overnight cultures were used to start fresh 250 ml cultures starting at a cell density of 0.05 OD 600 or less and grown to 0.1 OD 600 . Cells were stimulated with different concentrations of α-factor (Zymo Research, #Y1001) for 15 min, and cell lysates were prepared as described previously [33] . We used the same phospho-p44/42 MAP kinase antibody #9101 (Cell Signaling Technology) which cross-reacts with phosphorylated Kss1 or Fus3 MAP kinases that are activated by α-factor. Analysis of yeast morphological phenotypes S. cerevisiae cells were grown overnight in either complete or selective (-His, -Leu) low-fluorescence medium to make a preculture. From the preculture, fresh 3 ml cultures were started, beginning at 0.05 OD 600 or less cell density and grown at 30 °C with shaking up to 0.1 OD 600 . Cultures were treated with different concentrations of α-factor pheromone (Zymo Research #Y1001) and further incubated at 30 °C with shaking. To avoid heterogeneities from different stages of the cell cycle, α-factor-treated cells were incubated for 3 to 4 h before taking the images. For image acquisition by microscopy, 96-well optical quality clear bottom plates (NUNC) were used. Differential interference contrast images were acquired on a Nikon eclipse TE2000-U inverted microscope connected to a CoolSNAP CCD camera using a ×60 differential interference contrast H Plan APO oil objective. Numbers of cells showing different morphologies (axial budding, bipolar budding, cell cycle arrest and shmooing) were counted by eye following treatment of cells with pheromone α-factor [33] . For each condition, 500 to 700 cells were counted. Bcy1 mutagenesis and mutant analyses Conserved residues of the 'Reggai peptide' of human RIIβ (protein sequence accession number: NP_002727 ) were mutated in the sequence of the yeast regulatory subunit Bcy1 (protein sequence accession number: P07278 ). We mutated aspartic acid (D308) and glutamic acid (E317) to alanine (see Fig. 5b ). Mutagenesis was carried out using standard site-directed mutagenesis (Quikchange Site-Directed Mutagenesis Kit; Stratagene) following the manufacturer's instructions. The S.cerevisiae expression plasmid p415 (ADH promoter) bearing mutated bcy1 (=Bcy1*) was transformed into the bcy1Δ MAT a strain for analysis of MAPK activation and morphological responses as described above [33] . The R luc PCA [29] assay and the OyCD PCA [60] is performed as described previously. How to cite this article: Stefan, E. et al . PKA regulatory subunits mediate synergy among conserved G-protein-coupled receptor cascades. Nat. Commun. 2:598 doi: 10.1038/ncomms1605 (2011).